Telomerase stimulates ribosomal DNA transcription under hyperproliferative conditions In addition to performing its canonical function, Telomerase Reverse Transcriptase (TERT) has been shown to participate in cellular processes independent of telomerase activity. Furthermore, although TERT mainly localizes to Cajal bodies, it is also present within the nucleolus. Because the nucleolus is the site of rDNA transcription, we investigated the possible role of telomerase in regulating RNA polymerase I (Pol I). Here we show that TERT binds to rDNA and stimulates transcription by Pol I during liver regeneration and Ras-induced hyperproliferation. Moreover, the inhibition of telomerase activity by TERT- or TERC-specific RNA interference, the overexpression of dominant-negative-TERT, and the application of the telomerase inhibitor imetelstat reduce Pol I transcription and the growth of tumour cells. In vitro , telomerase can stimulate the formation of the transcription initiation complex. Our results demonstrate how non-canonical features of telomerase may direct Pol I transcription in oncogenic and regenerative hyperproliferation. Telomerase reverse transcriptase (TERT) is the rate-limiting component of the telomerase enzyme. Its canonical function is the elongation of telomeric DNA that is essential for all proliferating cells, including stem cells. Telomerase activity is suppressed in most human adult cells, but enhanced telomerase activity is detectable in the vast majority of human cancers, emphasizing its role in tumorigenesis. This process is mainly thought to occur through the stabilization of telomere length to overcome cellular crisis. There is accumulating evidence that telomerase may also contribute to tumorigenesis via mechanisms independent of telomere length. One interesting study demonstrated that a TERT construct that is incapable of telomere elongation induces transformation of an immortal telomerase-negative cell line in an oncogenic Ras-transfected background [1] . The molecular basis of these findings is still poorly understood, and extratelomeric functions of telomerase are the subject of intense debate [2] . Recent studies provided some insight into the mechanisms by which TERT may contribute to tumorigenic conversion of cells that extend beyond its canonical function. These studies demonstrated that telomerase can act as a transcriptional co-activator to regulate the Wnt pathway or can directly regulate NF-κB-dependent transcription [3] , [4] . Although telomerase mainly localizes to Cajal bodies [5] , distinct telomerase functions have been described in the cytoplasm, nucleolus, nucleus and mitochondria [6] , [7] , [8] . Notably, a recent report identified a nucleolar localization signal in TERT [9] . Interestingly, the nucleolar localization of TERT appears to be unrelated to its telomerase function [10] . Nucleoli are the sites of ribosomal biogenesis, and the key step in ribosomal biogenesis is transcription of rDNA by Pol I. This enzyme transcribes a precursor 47S rRNA transcript from the tandemly repeated rDNA locus, which is present in 530 copies per cell. This transcript is processed to generate the 18S, 5.8S and 28S rRNAs, which are the most abundant RNAs in the cell and serve structural and catalytic functions in the ribosomes. Transcription by Pol I comprises up to 70% of the total transcription in a growing cell and is dysregulated during tumorigenesis. Here, we show that telomerase binds the rDNA promoter and coding regions and stimulates transcription by Pol I in a proliferation-dependent manner. Moreover, inhibition of telomerase by short hairpin RNA (shRNA)-mediated knockdown of TERT, by the overexpression of dominant-negative (DN)-TERT, by short interfering RNA (siRNA) against TERC or by the telomerase inhibitor imetelstat reduces Pol I transcription and proliferation. These results indicate that telomerase acquires novel features upon the transition from resting to proliferating cells, and studying these changes may contribute to the understanding of the contribution of telomerase to tumorigenesis. Telomerase binds to rDNA First, we transfected human embryonic kidney (HEK) cells with haemagglutinin-tagged (HA-tagged) TERT and performed chromatin-immunoprecipitation (ChIP) analysis with antibodies specific for HA. As a positive control, we immunoprecipitated Pol I with an antibody directed against RPA135, one of the Pol I subunits. Antibodies against Pol I could precipitate chromatin-harbouring sequences of the rDNA promoter and the coding region but not of the intergenic spacer of the rDNA. Importantly, the rDNA promoter and all tested internal sequences, excluding the intergenic spacer, were identified with the HA-specific antibody targeting HA-TERT ( Fig. 1a ). In a control experiment, chromatin from non-transfected HEK cells was precipitated with an anti-HA antibody and did not yield rDNA sequences. We were able to amplify the region containing the TCF binding element 2 of the c-myc promoter, as reported by Park et al . [3] , whereas the 3′ untranslated region was not bound by HA-TERT ( Supplementary Fig.1b ). These results demonstrate the specificity of TERT–DNA interactions. 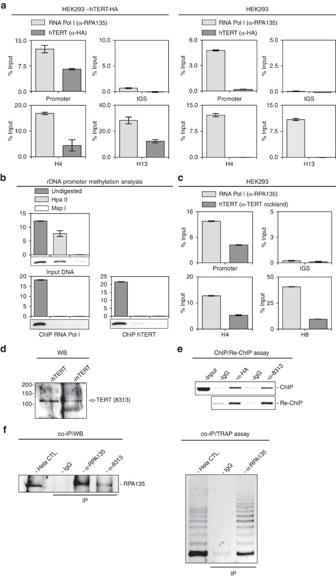Figure 1: Telomerase binds to promoter and internal regions of active rDNA. (a) HEK cells were transfected with HA-tagged TERT and subjected to ChIP experiments with the indicated antibodies and qPCR. As a control, the same experiment was performed with chromatin from non-transfected cells (IGS, intergenic spacer; H4, H8, H13, internal primers). Two representative internal gene sequences are shown. (b) The chromatin-immunoprecipitated DNA was digested by the indicated enzymes, and the rDNA promoter was detected by semiquantitative PCR and qPCR. (c) Endogenous TERT binds to rDNA. Chromatin from HEK cells was precipitated with the indicated antibodies (α-TERT (Rl), antibody from Rockland). (d) Western blot analysis with purified human and mouse TERT and AB8313. (e) ChIP-re-ChIP experiment with chromatin from HA-TERT-transfected HEK cells showing that the HA and 8313 antibodies both recognize a protein that binds the rDNA promoter. (f) Telomerase associates with Pol I. Coimmunoprecipitation of Pol I with anti-TERT AB8313 and an IP-TRAP assay with an anti-Pol I antibody. All panels are representative of at least three independent experiments. Error bars: s.e.m. Figure 1: Telomerase binds to promoter and internal regions of active rDNA. ( a ) HEK cells were transfected with HA-tagged TERT and subjected to ChIP experiments with the indicated antibodies and qPCR. As a control, the same experiment was performed with chromatin from non-transfected cells (IGS, intergenic spacer; H4, H8, H13, internal primers). Two representative internal gene sequences are shown. ( b ) The chromatin-immunoprecipitated DNA was digested by the indicated enzymes, and the rDNA promoter was detected by semiquantitative PCR and qPCR. ( c ) Endogenous TERT binds to rDNA. Chromatin from HEK cells was precipitated with the indicated antibodies (α-TERT (Rl), antibody from Rockland). ( d ) Western blot analysis with purified human and mouse TERT and AB8313. ( e ) ChIP-re-ChIP experiment with chromatin from HA-TERT-transfected HEK cells showing that the HA and 8313 antibodies both recognize a protein that binds the rDNA promoter. ( f ) Telomerase associates with Pol I. Coimmunoprecipitation of Pol I with anti-TERT AB8313 and an IP-TRAP assay with an anti-Pol I antibody. All panels are representative of at least three independent experiments. Error bars: s.e.m. Full size image Approximately 50% of the rDNA copies of a cell are actively transcribed; the other copies are epigenetically silenced by promoter methylation. To determine whether TERT binds the active rDNA copies, the precipitated chromatin was digested with a methylation-sensitive enzyme (HpaII) or a methylation-insensitive enzyme (MspI), and the rDNA promoter was subsequently amplified. HpaII treatment resulted in complete digestion of the chromatin precipitated by the Pol I antibody, indicating that Pol I only binds to unmethylated promoters. This result also occurred for the HA-precipitated chromatin ( Fig. 1b ). These results demonstrated that TERT binds the active fraction of the rDNA. Moreover, precipitating chromatin from non-transfected HEK cells with an established commercially available anti-TERT antibody [11] revealed that endogenous TERT binds the rDNA promoter and internal gene sequences ( Fig. 1c ). Together, these experiments indicate that telomerase is able to bind promoter and coding regions of rDNA. We characterized a newly generated antibody raised against a motif conserved between mouse and human TERT (AB8313). The specificity of this antibody was proven by western blot analysis with purified and enriched human and mouse TERT ( Fig. 1d ), by ChIP-re-ChIP experiments with chromatin from HA-TERT-transfected HEK cells ( Fig. 1e ), by the precipitation of the c-myc TCF binding element 2 site, by peptide competition with human and mouse chromatin and by IP-TRAP experiments with human and mouse nuclear extracts ( Supplementary Figs 1b,d and 2b ). To analyse whether RNA polymerase I and telomerase interact directly with each other, we performed coimmunoprecipitation experiments. As shown in Fig. 1f , the telomerase antibody precipitated substantial amounts of RNA polymerase I, and conversely, the RNA polymerase I antibody precipitated telomerase from nuclear extracts. These data indicate that the catalytic subunit of telomerase binds the active fraction of the rDNA and associates with RNA polymerase I. Telomerase binds rDNA under hyperproliferative conditions Binding of telomerase to rDNA was assessed under two physiological conditions. First, we addressed the binding activity of telomerase during cellular transformation. For this purpose, we used two experimental systems: (i) normal mouse liver tissue versus hepatocellular carcinoma tissue, because high telomerase activity can be detected in both samples [12] and (ii) IMR90 TERT-immortalized normal human fibroblasts, which contain the SV40 small- and large-T antigens (IMR90-hTERT-ST-LT), versus the transformed IMR90-hTERT-ST-LT cell line containing oncogenic Ras (RasV12). Notably, telomerase activity of these tissues and cell lines was comparable; however, we detected binding of TERT to rDNA exclusively in tumour cells and transformed cells ( Fig. 2a ). In addition, telomerase exhibited strong binding to rDNA in human hepatocellular carcinoma cells ( Supplementary Fig. 2a ). The specificity of the TERT antibody was further confirmed by telomerase binding to telomere sequences in dot blot and quantitative PCR (qPCR) analyses with chromatin-immunoprecipitated DNA from normal mouse liver and mouse liver tumours. Neither sample showed Pol I binding to telomeres, whereas telomerase exhibited strong binding to telomere ends in the tumour tissue but not in the normal mouse liver sample ( Fig. 2b ). Note that telomerase is recruited to telomere ends during the S-phase to function in telomere elongation [7] , [13] , [14] . Thus, telomere binding of telomerase can only be detected in liver tumours containing highly proliferative cells and not in normal livers containing resting cells, despite comparable levels of telomerase in both mouse samples (see Fig. 2a ). Second, to analyse whether TERT binding to rDNA is restricted to transformed cells and to better understand telomerase activity at the rDNA locus in vivo , we performed partial hepatectomies (PH) on the mice. PH triggers up to 80% of the resting, telomerase-positive hepatocytes in mice to enter the cell cycle and actively replicate [15] . Mice were subjected to PH and killed at different time points, and rDNA transcription and the binding kinetics of telomerase to rDNA were monitored ( Fig. 2c ). The association of telomerase with rDNA was detected as soon as 12 h after hepatectomy, and it peaked at 3 days post PH. After 10 days post PH, no significant rDNA could be precipitated with the telomerase antibody AB8313. Notably, endogenous telomerase activity is not significantly altered in regenerating liver [15] . Thus, rDNA occupancy of telomerase is a feature of proliferating hepatocytes. Pol I activity was increased threefold by PH and remained elevated until 10 days after PH, indicating that Pol I activity might not depend on telomerase binding to the rDNA ( Fig. 2d ). 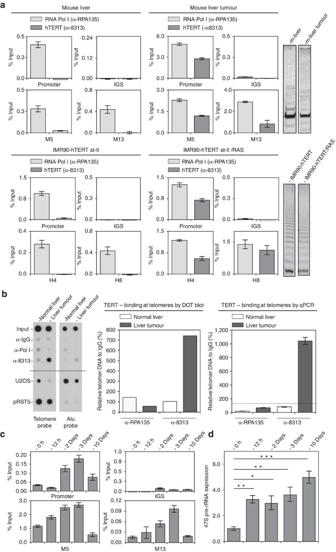Figure 2: Growth-dependent binding of telomerase to rDNA. (a) Quantitative PCR following ChIP experiments on the indicated tissues using antibodies against Pol I and telomerase (8313) demonstrating the growth signal dependence of the binding of TERT to rDNA. (b) Telomerase binds telomeric regions in tumour cells. Dot blot and qPCR analyses following ChIP experiments using the indicated antibodies from mouse liver/mouse liver tumour chromatin. Two amounts of U2OS genomic DNA or a plasmid harbouring telomeric sequences (pRST5) served as hybridization controls. (c) Binding dynamics of telomerase to the rDNA after PH. qPCR on chromatin harvested at the indicated time points after surgery immunoprecipitated using AB8313. Bars: s.e.m.. (d) Pol I transcription stimulation after PH. Quantitative PCR analysis of the 47S pre-rRNA synthesis at the indicated time points.n=3. (Pvalues: **=0.0067, *=0.0101, **=0.0025, ***=0.001, pairedt-test, two-tailed). All panels are representative of at least three independent experiments. Bars: s.e.m. Figure 2: Growth-dependent binding of telomerase to rDNA. ( a ) Quantitative PCR following ChIP experiments on the indicated tissues using antibodies against Pol I and telomerase (8313) demonstrating the growth signal dependence of the binding of TERT to rDNA. ( b ) Telomerase binds telomeric regions in tumour cells. Dot blot and qPCR analyses following ChIP experiments using the indicated antibodies from mouse liver/mouse liver tumour chromatin. Two amounts of U2OS genomic DNA or a plasmid harbouring telomeric sequences (pRST5) served as hybridization controls. ( c ) Binding dynamics of telomerase to the rDNA after PH. qPCR on chromatin harvested at the indicated time points after surgery immunoprecipitated using AB8313. Bars: s.e.m.. ( d ) Pol I transcription stimulation after PH. Quantitative PCR analysis of the 47S pre-rRNA synthesis at the indicated time points. n =3. ( P values: **=0.0067, *=0.0101, **=0.0025, ***=0.001, paired t -test, two-tailed). All panels are representative of at least three independent experiments. Bars: s.e.m. Full size image Telomerase stimulates Pol I transcription To elucidate the effect of TERT on Pol I transcription, we transfected IMR90-ST-LT cells with constant levels of a Pol I reporter vector harbouring the human rDNA promoter upstream of an rDNA sequence with increasing amounts of TERT vector. Reporter transcription was quantified by qPCR and indicated rDNA promoter activity. Increasing amounts of TERT in the absence of Ras repressed Pol I transcription in a dose-dependent manner ( Fig. 3a ). Importantly, transfecting cells with increasing amounts of TERT in the presence of Ras resulted in a fourfold stimulation of rDNA reporter transcription ( Fig. 3b ). Thus, TERT stimulates the key step of ribosomal biogenesis, transcription of RNA polymerase I, in a growth signal-dependent manner. 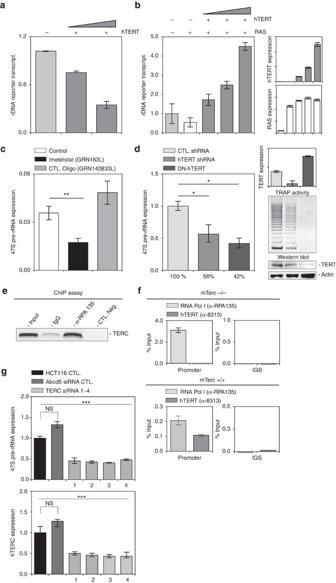Figure 3: Telomerase stimulates rDNA transcription. (a) qPCR analysis of rDNA reporter transcription after co-transfection with increasing amounts of TERT in IMR90-ST-LT cells. (b) Analysis of transcription of the rDNA reporter plasmid after co-transfection of TERT and RAS in IMR90-ST-LT cells.RASandTERTexpression levels were monitored by qPCR. Bars: s.e.m. (c) The telomerase inhibitor imetelstat inhibits Pol I transcription. IMR90-ST-LT-RAS/TERT cells were treated for 96 h with 5 μM of imetelstat or control oligo. RNA was harvested, and the synthesis of the 47S rRNA precursor was analysed by qPCR (Pvalue: 0.0016, unpairedt-test, two-tailed). (d) Knockdown of telomerase reduces Pol I transcription. HCT116 cells were transfected with control shRNA, TERT-shRNA or a DN-TERT construct. After antibiotic selection, 47S pre-rRNA and telomerase expression levels were monitored by qPCR. Telomerase activity was analysed by a TRAP assay, and TERT protein expression was analysed by western blotting (antibody: Rockland;Pvalues: 0.0253, 0.0159, unpairedt-test, two-tailed;n=3. Bars: s.e.m.). (e) TERC co-precipitates with Pol I antibodies from HEK chromatin. Chromatin-immunoprecipitated material was reverse transcribed and analysed with TERC-specific primers. (f) No binding of telomerase to rDNA in liver tumour cells from Terc−/− mice. ChIP analysis with anti-Pol I and anti-TERT-specific antibodies and the indicated primers. (g) siRNA against TERC reduces Pol I transcription. HCT116 cells were transfected with two controls and four anti-Terc siRNAs, and 47S and Terc expression levels were monitored by qPCR (P<0.0001, unpairedt-test, two-tailed). All panels are representative of at least three independent experiments. Error bars: s.e.m. Figure 3: Telomerase stimulates rDNA transcription. ( a ) qPCR analysis of rDNA reporter transcription after co-transfection with increasing amounts of TERT in IMR90-ST-LT cells. ( b ) Analysis of transcription of the rDNA reporter plasmid after co-transfection of TERT and RAS in IMR90-ST-LT cells. RAS and TERT expression levels were monitored by qPCR. Bars: s.e.m. ( c ) The telomerase inhibitor imetelstat inhibits Pol I transcription. IMR90-ST-LT-RAS/TERT cells were treated for 96 h with 5 μM of imetelstat or control oligo. RNA was harvested, and the synthesis of the 47S rRNA precursor was analysed by qPCR ( P value: 0.0016, unpaired t -test, two-tailed). ( d ) Knockdown of telomerase reduces Pol I transcription. HCT116 cells were transfected with control shRNA, TERT-shRNA or a DN-TERT construct. After antibiotic selection, 47S pre-rRNA and telomerase expression levels were monitored by qPCR. Telomerase activity was analysed by a TRAP assay, and TERT protein expression was analysed by western blotting (antibody: Rockland; P values: 0.0253, 0.0159, unpaired t -test, two-tailed; n =3. Bars: s.e.m.). ( e ) TERC co-precipitates with Pol I antibodies from HEK chromatin. Chromatin-immunoprecipitated material was reverse transcribed and analysed with TERC-specific primers. ( f ) No binding of telomerase to rDNA in liver tumour cells from Terc−/− mice. ChIP analysis with anti-Pol I and anti-TERT-specific antibodies and the indicated primers. ( g ) siRNA against TERC reduces Pol I transcription. HCT116 cells were transfected with two controls and four anti-Terc siRNAs, and 47S and Terc expression levels were monitored by qPCR ( P <0.0001, unpaired t -test, two-tailed). All panels are representative of at least three independent experiments. Error bars: s.e.m. Full size image We next examined whether inhibition of endogenous telomerase would affect Pol I transcription. First, we used imetelstat (GRN163L) to inhibit telomerase activity and monitored Pol I activity. As depicted in Fig. 3c , imetelstat, but not the control oligo (GRN140833L), severely affected Pol I transcription, indicating that half of Pol I activity in transformed cells is due to stimulation by telomerase. Furthermore, we transfected HCT116 cells with a TERT-specific shRNA or with a DN-TERT mutant (DN-TERT) and monitored Pol I transcription. The expression levels of endogenous TERT and DN-TERT were monitored by qPCR and western blotting, demonstrating that DN-TERT expression is followed by the degradation of endogenous TERT protein [16] . TERT-shRNA, and to a greater extent DN-TERT, significantly reduced telomerase activity, as demonstrated in the TRAP assay ( Fig. 3d ). Strikingly, the inhibition of telomerase activity by TERT-shRNA or DN-TERT reduced Pol I activity as measured by endogenous 47S transcription to 56% or 42%, respectively, of the control level. Thus, repressing telomerase activity directly reduces rDNA transcription. Telomere length was not significantly affected during this short period of treatment ( Supplementary Fig. 3b ), indicating that telomere elongation and stimulation of rDNA transcription by telomerase are not causally linked. Taken together, the dose-dependent stimulation of Pol I by transfection with TERT and the decrease in Pol I transcription by the inhibition of telomerase activity strongly support the hypothesis that TERT and telomerase directly regulate transcription by Pol I. We next investigated whether only TERT binds rDNA or whether TERC can also be coprecipitated with Pol I chromatin. We reverse transcribed the immunoprecipitated chromatin (to generate cDNA for the RNA component of telomerase) and were able to amplify TERC from Pol I chromatin, indicating that telomerase binds in a complex to the rDNA ( Fig. 3e ). This observation is consistent with previous reports showing TERC localization in the nucleoli of HeLa cells [7] , [17] . Moreover, when liver tumour cells derived from Terc−/− mice [18] were subjected to ChIP analysis, no binding of TERT to the rDNA promoter was detectable, arguing that the presence of TERC in the telomerase complex is necessary for the association of TERT with the rDNA ( Fig. 3f ). In addition, a reduction in TERC expression by siRNA transfection in HCT116 cells impaired RNA polymerase I transcription—as monitored by transcription of the 47S pre-rRNA precursor—indicating that influencing ribosomal biogenesis requires both telomerase subunits ( Fig. 3g ). These findings demonstrate for the first time a novel telomere length-independent role for telomerase in regulating Pol I-dependent gene transcription, which has implications for cellular proliferation. Telomerase stimulates initiation at the rDNA promoter Next, in vitro transcription experiments were used to gain mechanistic insights into the action of telomerase at the rDNA promoter. Template-immunoprecipitation experiments [19] exploring the kinetics of telomerase at the rDNA promoter after the initiation of transcription revealed that telomerase does not leave the rDNA promoter with Pol I but stays bound to the template during transcription ( Fig. 4a ). ChIP experiments involving the inhibition of telomerase by shRNA or the expression of a DN-TERT showed reduced promoter occupancy of the rDNA by telomerase ( Fig. 4b ). This reduction in promoter occupancy may have caused the reduction in the in vitro Pol I transcription activity of nuclear extracts collected from the treated HCT116 cells. In addition to multiple-round transcription, single-round transcription was also severely affected by the repression of telomerase. Promoterless transcription and run-on transcription by Pol I were not reduced by telomerase repression, indicating that binding of telomerase to internal positions on the rDNA might not directly influence transcription elongation ( Fig. 4c , Supplementary Fig. 3b ). Next, we performed reconstitution experiments with purified TERT expressed in various cell types. The reconstitution of in vitro RNA polymerase I transcription was only successful when TERT was expressed in Terc-competent cells (derived from a telomerase-positive mouse liver tumour [18] ), whereas expression of TERT in Terc−/− cells (derived from a Terc-negative mouse liver tumour [18] ) did not stimulate Pol I transcription ( Fig. 4d ). Reconstitution experiments with TERT expressed and purified in HEK cells confirmed that telomerase stimulates initiation complex formation at the rDNA promoter, as demonstrated by the stimulation of single-round transcription by the addition of telomerase ( Fig. 4e ). The signal strength in single-round transcription is directly proportional to the number of initiation complexes formed at the promoter: every initiation complex yields one molecule of RNA because re-initiation is impaired by the addition of sarkosyl after the start of transcription [19] . Moreover, template-immunoprecipitation experiments titrating telomerase to TERT-shRNA-derived nuclear extracts revealed that more RNA polymerase I complexes are formed at the rDNA promoter in the presence of telomerase ( Fig. 4f ). Taken together, these data imply that telomerase increases the number of active initiation complexes at the rDNA promoter and remains at the promoter during transcription. 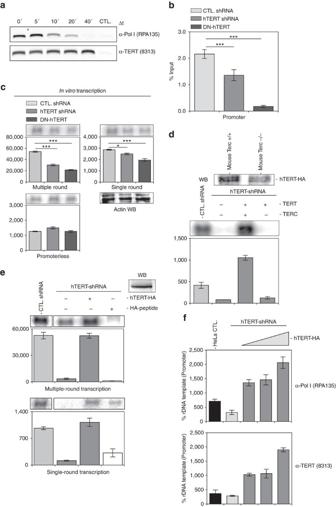Figure 4: Telomerase stimulates initiation complex formation at the rDNA promoter. (a) A template-immunoprecipitation experiment revealed that telomerase does not leave the rDNA promoter during transcription. After pre-incubation of HeLa nuclear extract with rDNA template, thein vitrotranscription reaction was started by the addition of nucleotides and stopped after the indicated time points by cross-linking with formaldehyde. Pol I and telomerase were precipitated with antibodies, and the associated template was detected by PCR. (b) Inhibition of telomerase reduces rDNA promoter occupancy of telomerase in HCT116 cells. ChIP experiments with telomerase-specific antibodies and analysis of TERT binding to the rDNA promoter (P<0.0001, unpairedt-test, two-tailed). (c)In vitrotranscription of Pol I with nuclear extracts of shRNA-treated HCT116 cells. A representative RNA gel electrophoresis image is shown. Actin served as a loading control for western blotting (Pvalues: multiple round:P<0.0001; single round: 0.0169, 0.0003, unpairedt-test, two-tailed). (d) Purified TERT from Terc −/− cells does not stimulatein vitrotranscription by Pol I. HA-TERT was expressed in competent mouse liver cells or those lacking Terc, purified and used forin vitrotranscription. (e) Reconstitution of Pol I single-round transcription with purified telomerase (western blot with anti-HA) demonstrates that telomerase stimulates initiation complex formation at the rDNA promoter. Quantification of data from a representative experiment was performed through phosphorimager analysis (Fujifilm fla-3000) and the use of an AIDA Image Analyzer. (f) Template-immunoprecipitation experiment showing that titration of purified telomerase to nuclear extract of TERT-repressed cells enhances binding of Pol I to the rDNA promoter. All panels are representative of at least three independent experiments. Bars: s.e.m. Figure 4: Telomerase stimulates initiation complex formation at the rDNA promoter. ( a ) A template-immunoprecipitation experiment revealed that telomerase does not leave the rDNA promoter during transcription. After pre-incubation of HeLa nuclear extract with rDNA template, the in vitro transcription reaction was started by the addition of nucleotides and stopped after the indicated time points by cross-linking with formaldehyde. Pol I and telomerase were precipitated with antibodies, and the associated template was detected by PCR. ( b ) Inhibition of telomerase reduces rDNA promoter occupancy of telomerase in HCT116 cells. ChIP experiments with telomerase-specific antibodies and analysis of TERT binding to the rDNA promoter ( P <0.0001, unpaired t -test, two-tailed). ( c ) In vitro transcription of Pol I with nuclear extracts of shRNA-treated HCT116 cells. A representative RNA gel electrophoresis image is shown. Actin served as a loading control for western blotting ( P values: multiple round: P <0.0001; single round: 0.0169, 0.0003, unpaired t -test, two-tailed). ( d ) Purified TERT from Terc −/− cells does not stimulate in vitro transcription by Pol I. HA-TERT was expressed in competent mouse liver cells or those lacking Terc, purified and used for in vitro transcription. ( e ) Reconstitution of Pol I single-round transcription with purified telomerase (western blot with anti-HA) demonstrates that telomerase stimulates initiation complex formation at the rDNA promoter. Quantification of data from a representative experiment was performed through phosphorimager analysis (Fujifilm fla-3000) and the use of an AIDA Image Analyzer. ( f ) Template-immunoprecipitation experiment showing that titration of purified telomerase to nuclear extract of TERT-repressed cells enhances binding of Pol I to the rDNA promoter. All panels are representative of at least three independent experiments. Bars: s.e.m. Full size image Inhibition of Telomerase or Pol I retards proliferation Ribosomal biogenesis is a prerequisite for growth and proliferation, and telomerase acts as a growth-promoting factor [20] , [21] , [22] . Thus, we investigated whether the inhibition of Pol I transcription by knockdown of TERT influences cellular proliferation and analysed the increase in the number of HCT116 cells stably transfected with the hTERT-specific shRNA or with the DN-hTERT construct. As shown in Fig. 5a , knockdown of TERT is followed by strong inhibition of cellular proliferation. Reduced Pol I transcription following TERT inhibition results in a decrease in mature ribosomal RNA subunits as evaluated by qPCR ( Fig. 5a ). These results indicate that the level of transcription by Pol I may be a critical factor affecting cell cycle dynamics. Previous reports showed that the rate of ribosome biogenesis controls cell cycle progression [23] , [24] . To address this hypothesis, HCT116 cells were subjected to specific RNA polymerase I inhibition by the small molecule inhibitor CX5461 (ref. 25 ), and Pol I transcription, proliferation dynamics and ribosomal content were analysed. Specific inhibition of Pol I transcription severely reduced the proliferation rate of the cells and the ribosomal content ( Fig. 5b ). These results suggest that the proliferation rate and the cell cycle dynamics are determined by the rate of rRNA synthesis by Pol I and that the telomerase complex influences the proliferation rate by stimulating rDNA transcription. 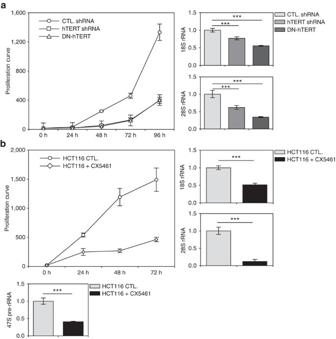Figure 5: Proliferation of cells upon the inhibition of telomerase or Pol I. (a) Telomerase inhibition retards proliferation and ribosomal biogenesis. HCT116 cells stably transfected with the indicated shRNA constructs were monitored for proliferation and by qPCR for their mature rRNA content (18S:P<0.0001; 28S:P=0.0004,P<0.0001, unpairedt-test, two-tailed). (b) Specific inhibition of Pol I reduces proliferation and ribosomal rRNA content. In this assay, 150 nm of the small molecule inhibitor CX5461 was added to the medium of HCT116 cells, and cells were counted at the indicated time points. RNA was harvested and analysed by qPCR with the indicated primers (18S:P<0.0001, 28S:P=0.0003, 47S:P<0.0001, unpairedt-test, two-tailed). Experiments were performed in triplicate. Bars: s.e.m. Figure 5: Proliferation of cells upon the inhibition of telomerase or Pol I. ( a ) Telomerase inhibition retards proliferation and ribosomal biogenesis. HCT116 cells stably transfected with the indicated shRNA constructs were monitored for proliferation and by qPCR for their mature rRNA content (18S: P <0.0001; 28S: P =0.0004, P <0.0001, unpaired t -test, two-tailed). ( b ) Specific inhibition of Pol I reduces proliferation and ribosomal rRNA content. In this assay, 150 nm of the small molecule inhibitor CX5461 was added to the medium of HCT116 cells, and cells were counted at the indicated time points. RNA was harvested and analysed by qPCR with the indicated primers (18S: P <0.0001, 28S: P =0.0003, 47S: P <0.0001, unpaired t -test, two-tailed). Experiments were performed in triplicate. Bars: s.e.m. Full size image Telomerase is repressed in most human adult tissues, but it can be detected in cells with high proliferation capacity, such as activated B- and T-cells and stem cells. In addition, reactivation of telomerase is observed in approximately 90% of human tumours. Initially, telomerase activity was thought to be required solely to prevent telomere shortening. Recent data support the emerging idea that hTERT/telomerase possesses pro-tumorigenic activities that extend beyond its classical role in telomere elongation. Interestingly, in mouse tumours originating from telomerase-positive tissues, an increase in telomerase activity has been observed, and overexpression of telomerase supports tumour formation in mouse tissues with long telomeres, indicating that telomerase has functions in tumorigenesis that are independent of telomere lengthening [1] , [26] , [27] , [28] . Here, we describe a novel non-canonical function of telomerase. We show that telomerase binds to rDNA and stimulates transcription in a regenerative- or growth signal-dependent manner. Our results are consistent with recent findings on the binding of TERT to extratelomeric motifs, suggesting a novel function of telomerase as a transcriptional co-regulator of Wnt or NF-κB signalling [3] , [4] . TERT binding to the TCF3 binding sites was observed in HeLa cells and proliferating gut epithelium [3] . Thus, the binding dynamics of TERT to the TCF sites may also be influenced by oncogenes or growth signals, as shown in our study. Human cancer cells have a rapid and defined growth-inhibitory response to telomerase inhibition independent of bulk telomere shortening [29] . Imetelstat, a potent novel antitumour drug, targets telomerase and depletes cancer stem cells in a telomere lengthening-independent manner [30] . This result is consistent with our observations that the inhibition of telomerase activity by either shRNA or DN-hTERT inhibits ribosomal biogenesis and cellular proliferation. It is tempting to speculate that the reduction in ribosomal biogenesis due to altered cell cycle dynamics [23] , [24] contributes to the growth inhibition observed after telomerase depletion in cancer cells. Using a reporter assay, we show oncogene/growth signal-dependent stimulation of Pol I transcription by TERT. The reporter experiments by Park et al . [3] demonstrating a stimulatory effect of TERT on genes of the Wnt pathway were performed in tumour cells; thus, they do not exclude the possibility that the described effects of TERT are also dependent on a tumour environment. Moreover, our study shows a telomerase activity dependence of the stimulatory effect of telomerase on Pol I transcription, as measured by a TRAP assay. The DN-TERT mutant, which carries a point mutation inactivating the telomere elongation capacity [31] , does not stimulate Pol I activity but rather represses rDNA transcription ( Fig. 3d ), possibly by the export and degradation of the endogenous telomerase [16] . This result, together with results on the inhibition by imetelstat and the dependence of rDNA binding and the stimulation of Pol I transcription on the presence of TERC, demonstrates that the enzymatic activity of telomerase is required for stimulating rDNA transcription. In vitro transcription experiments showed that telomerase with a C-terminal HA-tag, which possesses enzymatic activity but cannot elongate telomeres [32] , still stimulates rDNA transcription ( Supplementary Fig. 3a ). This result indicates that an enzymatic activity of telomerase other than the canonical activity may be required for the positive effect on rDNA transcription. Because telomerase is also active at the telomeres during replication in proliferating cells, we conclude that enzymatically active telomerase is important for both telomere elongation and Pol I transcription, but our results provide no evidence of an epistatic relationship between these two processes. Taken together, our data indicate the existence of a novel mechanism associated with telomerase enzymatic activity. This function differs from previous findings describing telomere length- and telomerase-independent functions of hTERT [3] , [33] , [34] , [35] , [36] , [37] see also review in ref. 38 . Interestingly, Ghosh et al . [4] also found that functional telomerase is required to regulate NF-κB signalling. The authors observed that the telomerase holoenzyme is important for NF-κB-dependent gene expression. Moreover, the binding of telomerase to NF-κB-dependent genes and expression stimulation was markedly enhanced and rapidly activated by the addition of TNF-α. A recent report, however, showed that TERT can function independent of its enzymatic function to regulate the NF-κB-dependent transcription [37] . This discrepancy requires clarification in future studies. In our study, we observe non-oncogenic rDNA binding of telomerase when resting hepatocytes enter a proliferative mode. This observation may reflect a physiological response to an elevated need for ribosomes and is supported by the observation of Ghosh et al . [4] that the NF-κB pathway is dampened in telomerase-knockout animals, indicating a physiological role for telomerase in gene regulation in vivo. It is interesting that mice with a hypomorphic DKC1 (dyskeratosis congenita 1) mutant protein show dysregulated ribosome function [39] . DKC1, which is necessary for proper rRNA processing, is a part of the telomerase complex, and a subset of dyskeratosis congenita patients have mutations in TERT or TERC, the core components of telomerase. Thus, extratelomeric functions of telomerase may contribute to the pathology of dyskeratosis congenita. Although a final conclusion regarding the extratelomeric functions of telomerase is still elusive and unresolved, our data support the notion that the nucleolar-localized telomerase stimulates rRNA transcription. Human cancer cells have a rapid and defined growth-inhibitory response to telomerase inhibition that is independent of bulk telomere shortening [29] . This observation is consistent with our observations that the inhibition of telomerase activity by either shRNA or DN-hTERT inhibits ribosomal biogenesis and the proliferation of tumour cells. Our results strengthen the hypothesis that a reduction in ribosomal biogenesis might contribute to the growth inhibition observed after telomerase depletion in cancer cells. We also provide the first mechanistic insight into the action of telomerase as a transcription factor: in vitro transcription assays show that TERT remains bound to the template during transcription and stimulates initiation complex formation at the rDNA promoter, implying that telomerase is able to recruit or stabilize the binding of Pol I initiation factors or the polymerase at the promoter. Because this feature depends on growth signals or proliferation, telomerase stabilises Pol I transcription initiation when there is a high demand for ribosomal transcription. In summary, these data indicate that telomerase acts as a transcription factor for Pol I. In addition, we show that the DNA-binding features of TERT are proliferation-dependent. Moreover, our data imply that by stimulating ribosomal biogenesis, telomerase influences cell cycle and proliferation dynamics. Antibody generation A mouse/human conserved peptide sequence (amino acids 568–581 for human TERT and amino acids 558–571 for mouse TERT) was chosen for the production of the anti-TERT antibody AB8313: FQKNRLFFYRKSVW C . The peptide was synthesized at the Heinrich-Pette Institute on an ABI peptide synthesizer (ABI 433 A), and purity was assessed by HPLC. The last amino acid, the underlined cysteine, is not part of the TERT sequence but was added for efficient conjugation to KLH (Keyhole Limpet Haemocyanin), and the first conjugate (500 μg conjugated peptide) was injected into two rabbits with Complete Freund’s Adjuvant (F5881, Sigma-Aldrich Co.). This injection was followed by two booster injections with Incomplete Freund’s Adjuvant (F5506, Sigma-Aldrich Co.), and all injections were conducted in the animal facility of the University Hospital of Hamburg (UKE, Hamburg, Germany). The third and final bleedings of both animals were pooled (~100 ml) and were affinity purified according to standard procedures. The production and purification of RPA135 was described in detail previously [19] . Antibodies For ChIP analysis, 2–4 μg of anti-HA antibody (Roche #11867423001) was used. The purification of overexpressed and tagged TERT was performed with anti-HA-agarose (Sigma-Aldrich Co. #A2095). Western blot detection of HA-TERT was performed using an anti-HA antibody (Cell Signaling #2367S) at a dilution of 1:1,000. Endogenous TERT was analysed with an anti-TERT antibody (Rockland #8006567625) at a dilution of 1:500. Western blot analysis of Pol I with anti-RPA135 was conducted with a dilution of 1:1,000, and analysis of purified h/mTERT was performed with Ab8313 using a dilution of 1:100. Chromatin-immunoprecipitation ChIP experiments were performed as described previously [19] . Briefly, cells or ground tissues were cross-linked by the addition of formaldehyde to a final concentration of 1% for 10 min, and the reaction was stopped by the addition of glycine (125 mM). Chromatin was fragmented by sonication. Fragment size was controlled by agarose gel electrophoresis. For this assay, 50 μl of chromatin, corresponding to 0.5–2 × 10 6 cells, was precleared with protein A agarose (Sigma-Aldrich Co.) and subjected to precipitation with 2–4 μg of antibody. After precipitation and sequential washing, cross-linked proteins were digested by incubation with elution buffer (TE buffer; 1% SDS) and Proteinase K for 2 h at 68 °C. DNA was extracted using the QIAquick Nucleotide Removal Kit (QIAGEN GmbH) and analysed by PCR. Statistical analysis of qPCR was performed according to Tukey’s multiple comparison test. ChIP-re-ChIP experiments: after the first immunoprecipitation and washes, protein-DNA complexes were eluted with 10 mM DTT and diluted before the addition of antibodies and protein A-Sepharose beads for the second immunoprecipitation. The primer sequences used for human and mouse rDNA amplification for semiquantitative and real-time PCR analyses were published by O’Sullivan [40] and are provided in the Supplementary Table 1 . Telomerase assay The telomere repeat amplification protocol was performed with a kit (TRAPeze, Chemicon) according to the manufacturer’s instructions. In brief, 100–250 ng of nuclear extract was incubated with the TRAP primer and nucleotides for telomerase extension for 30 min at 30 °C, followed by PCR amplification (30 cycles). Products were resolved with 12.5% polyacrylamide gel electrophoresis (PAGE) and visualized with SYBR green (Invitrogen). Cell culture, transfections and vectors HEK (293), IMR90 and HCT116 cells were cultivated in Dulbecco’s Modified Eagle Medium with 10% fetal bovine serum in the presence of antibiotics (penicillin/streptomycin). Transient transfection of HEK cells with HA-tagged TERT was performed using standard procedures with CaCl 2 . For stable expression, IMR90 cells were transduced with retroviral vectors (pBABE-Puro-hTERT, SV40-ST-LT-Ags and pBABE-bla-RasV12) according to standard protocols and selected with 0.5 μg ml −1 puromycin, 500 μg ml −1 G418 or 2 μg ml −1 blasticidin, respectively. Transient co-transfection experiments with hTERT-HA, HA-hTERT, RasV12 and a rDNA reporter pHrP 2 BH bearing the rDNA promoter and a piece of rDNA flanked by two termination sites (kind gift of I. Grummt) were performed with the Nucleofector device from Lonza according to the manufacturers’ protocol. After 48 h, RNA was extracted (RNeasy, Qiagen), reverse transcribed and analysed by PCR with the indicated primers. HCT116 cells were transfected with scrambled, TERT-shRNA or DN-TERT constructs by using Attractene (Qiagen) and were selected after 48 h by the addition of puromycin (0.5 μg ml −1 ). siRNA against Terc (Qiagen #GS7012) was transfected into HCT116 cells with HiPerFect (Qiagen) according to the manufacturer’s instructions. The mouse cell lines used for expression of telomerase with and without TERC were established in house (A.L.) The pBABE-bla-RasV12 vector expressing the constitutively active Ras mutant was generated by PCR amplification from the pWZL-Hygro-RasV12 vector (kindly provided by Scott Lowe). The pBABE-Puro-hTERT, pBABE-Puro-hTERT-HA, pWZL-HA-hTERT, pBABE-Puro-DN-hTERT and pBABE-neo largeT vectors were provided by R. Weinberg, and the hTERT-shRNA vector was a gift from William Hahn (Addgene Plasmid 10688). For knockdown of telomerase activity, a lentiviral vector harbouring hTERT-shRNA was used, and the cells were selected with puromycin (0.5 μg ml −1 ). Western blotting HCT116 cells were lysed in the presence of proteinase (complete, Roche) and phosphatase inhibitors (NaF, NaVO 3 , β-glycerophosphate), subjected to SDS–PAGE, and transferred to nitrocellulose. Purification of telomerase HEK (293) cells were transfected with pBABE-Puro-hTERT-HA and lysed after 48 h in a buffer containing NP-40. Each sample of 2.5 mg lysate was incubated with anti-HA-agarose beads (Sigma-Aldrich Co.) in the presence of protease inhibitors on a rotating wheel at 4 °C overnight. After three washes with AM300+0.1% NP-40, bound telomerase was eluted from the beads by incubation at 4 °C for 2 h in AM100 plus 0.5 μg μl −1 HA peptide and tested in western blot and in in vitro transcription. In vitro transcription The following templates were employed for specific in vitro transcription assays. The pHrP 2 plasmid, harbouring a human rDNA fragment spanning bases −411 to +375 relative to the transcription initiation site was linearized with EcoRI. The template for nonspecific in vitro transcription was a 267-bp fragment that was excised from pUC18 with NdeI and EcoRI. Briefly, incubation of 40 μg of nuclear extracts with 40 ng of template DNA was performed under standard transcription conditions in a volume of 25 μl (16 mM Tris–HCl (pH 8.0), 5 mM MgCl 2 , 0.2 mM EDTA, 80 mM KCl, 10% (v/v) glycerol, 0.66 mM each ATP, CTP and GTP, 12.5 μM UTP, and 1 μCi of [α- 32 P]UTP (800 Ci mmol −1 )). After incubation for 60 min at 30 °C, proteins were digested with 25 μl of Proteinase K Mix for 30 min at 40 °C, synthesized RNA was precipitated with 200 μl of ice cold 100% ethanol and 25 μl of 7.5 M ammonium acetate, washed with 100 μl 70% ethanol and resolved on 4% polyacrylamide gels. Gels are provided in Supplementary Fig. 4 . PH We used 8-week-old male wild-type mice with a C57BL/6 J background for PH. The mice were maintained in a pathogen-free environment and fed a standard diet. All mice were operated on in the morning (between 09:00 and 11:00) as described in ref. 41 . Mice were anaesthetized with ketamine (100 mg kg −1 body weight)/xylazine (10 mg kg −1 body weight) and subjected to 70% PH by surgically removing the left lateral, left median and right median lobes without disrupting the portal vein, biliary tract or gallbladder. The mice were euthanized at 12 h ( n =3), 48 h ( n =3), 72 h ( n =3) and 120 h ( n =3) after PH. Then, the liver lobes were snap-frozen in liquid nitrogen and stored at −80 °C until further analysis. Animal experiments were approved by the state government of Baden-Wuerttemberg (Protocol Number 35/9185.81-3/919). Template immunoprecipitation Each sample of 40 ng rDNA template (pHrP2 linearized with EcoRI) was centrifuged with 40 μg of the indicated nuclear extracts and 0.825 μmol guanine for 40 min at 30 °C and 350 r.p.m. The addition of sarcosyl (final concentration: 0.025%) and salmon sperm DNA (final concentration: 400 ng) ensured single-round transcription. Transcription was initiated by adding ribonucleotides and stopped after the indicated times by cross-linking proteins to the template with formaldehyde. Each sample was diluted with IP buffer and incubated with the indicated antibodies overnight at 4 °C. Isolation of precipitated complexes, washing steps, digestion of proteins and DNA extraction, as well as DNA amplification, were performed as described for the ChIP analysis. Statistics Each experiment was repeated at least three times. For the ChIP experiments in Fig. 2 , each experiment was performed with chromatin from either three different mouse livers or three different mouse liver tumours. Three different mice were used for each time point in the PH experiment ( Fig. 2 ). All statistical analyses were performed using GraphPad Prism (GraphPad Software, Inc., La Jolla, CA 92037, USA). Significant differences between transfection with control shRNA, hTERT-specific shRNA and the DN-TERT construct ( Fig. 3d ) were calculated using the t -test (unpaired, two-tailed). For the statistical analysis of the PH experiment, we used a paired t -test (two-tailed). How to cite this article : Gonzalez, O. G. et al . Telomerase stimulates ribosomal DNA transcription under hyperproliferative conditions. Nat. Commun. 5:4599 doi: 10.1038/ncomms5599 (2014).